Nucleic acid sensing by T cells initiates Th2 cell differentiation While T-cell responses are directly modulated by Toll-like receptor (TLR) ligands, the mechanism and physiological function of nucleic acids (NAs)-mediated T cell costimulation remains unclear. Here we show that unlike in innate cells, T-cell costimulation is induced even by non-CpG DNA and by self-DNA, which is released from dead cells and complexes with antimicrobial peptides or histones. Such NA complexes are internalized by T cells and induce costimulatory responses independently of known NA sensors, including TLRs, RIG-I-like receptors (RLRs), inflammasomes and STING-dependent cytosolic DNA sensors. Such NA-mediated costimulation crucially induces Th2 differentiation by suppressing T-bet expression, followed by the induction of GATA-3 and Th2 cytokines. These findings unveil the function of NA sensing by T cells to trigger and amplify allergic inflammation. Toll-like receptors (TLRs) sense pathogen-associated molecular patterns to initiate not only innate responses but also to help regulate T cell-mediated adaptive immune responses [1] , [2] . While some TLRs are expressed on the cell surface, NA-sensing TLRs such as TLR3, TLR7/8 and TLR9 are expressed in endosomal compartments, allowing specific recognition of endocytosed pathogens. Recent studies have shown that T cells also express TLRs and that TLR ligands can directly modulate T-cell responses. For example, TLR2 ligands directly promote proliferation of activated T cells [3] , [4] , modulate the proliferation and suppressive functions of CD4 + CD25 + regulatory T cells [5] , [6] , trigger Th1 effector functions independently of TCR stimulation [7] and modulate Th17 responses [8] . In addition, it has been reported that ligands for NA-sensing TLRs enhance IL-2 production and proliferation of anti-CD3 antibody (Ab)-stimulated T cells [9] , [10] and promote survival of activated T cells [11] , and further that the TLR8 ligand inhibits the suppressive function of regulatory T cells [12] . However, except for TLR2, very little is known about the molecular basis of the NA-sensing mechanisms and the functional consequences of NA-mediated costimulation in T cells. Naıve CD4 + T cells differentiate into various effector T helper (Th) cells such as Th1, Th2 and Th17 cells, which produce IFN-γ, IL-4/IL-5/IL-9/IL-13 and IL-17/IL-22, respectively [13] . While Th1 and Th17 cells exhibit protective functions against intracellular pathogens and extracellular bacteria/fungi, Th2 cells protect from helminthic infection. Contrary to these protective functions, the same Th subsets can play a role in disease pathogenesis: Th1 for inflammatory diseases, Th2 for allergic diseases and Th17 for autoimmune diseases. While TLR stimulation of antigen-presenting cells (APCs) results in the production of IL-12, which induces Th1 differentiation, Th2 development is induced by IL-4, but the cells responsible for the initial wave of IL-4 production needed to induce Th2 differentiation remain elusive [14] . In this study, we report that NA-induced costimulatory responses of CD4 + T cells are mediated independently of known NA sensors in innate immunity. We found that T cells take up NAs to induce costimulation and that the NA-mediated costimulation requires higher-order structure of the NAs by forming complexes with the antimicrobial peptides or with core histones. More importantly, costimulation of naive CD4 + T cell with NAs induces Th2 differentiation through the downregulation of T-bet and the upregulation of GATA-3 expression. Thus, NAs directly induce T-cell costimulation through a unique NA-sensing mechanism to trigger the initial IL-4 production for Th2 differentiation, which might be involved in triggering and amplification of allergic inflammation. TLR-independent NA-mediated costimulation of CD4 + T cells To elucidate the functional significance of NA stimulation, naive CD4 + T cells were stimulated with each TLR ligand. While none of the TLR ligands alone were able to induce cell proliferation or IL-2 production, proliferation and IL-2 production were selectively enhanced by Pam3 (TLR1/2), MALP-2 (TLR2/6), poly(I:C) (TLR3) and CpG-B (TLR9) with anti-CD3 stimulation ( Fig. 1a ). 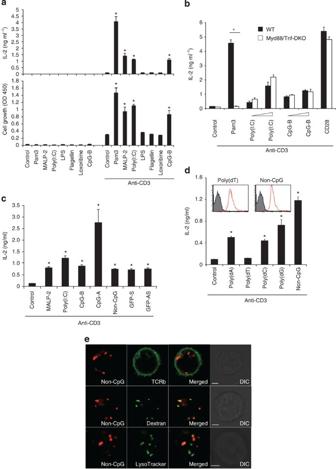Figure 1: DNA/RNAs are incorporated into and induce costimulation of CD4+T cells. (a) Naive CD4+T cells were cultured with indicated TLR ligands (Pam3: 5 μg ml−1, MALP-2: 5 μg ml−1, poly(I:C): 100 μg ml−1, Flagellin: 1 μg ml−1, Loxoribine: 100 μM, CpG-B: 5 μM) in the presence or absence of immobilized anti-CD3∈Ab (10 μg ml−1). After 48-hour incubation, IL-2 production and cell growth were assessed by ELISA and MTS assay, respectively. *P<0.05, Student’st-test (compared with anti-CD3 alone). (b) Naive CD4+T cells from WT orMyd88−/−Trif−/−mice were stimulated with the indicated TLR ligands or anti-CD28 (Clone: 37.51, 5 μg ml−1) in the presence of immobilized anti-CD3∈Ab. *P<0.05, Student’st-test (compared with WT cells treated with Pam3). (c,d) Naive CD4+T cells were stimulated with the indicated NAs (c) and ODNs (d) in the presence of immobilized anti-CD3∈Ab. These T cells were incubated with the Cy5-labelled ODNs at 37 °C for 90 min and ODN uptake was determined by flow cytometry (d, upper). *P<0.05, Student’st-test (compared with anti-CD3 alone). (e) Naive CD4+T cells were incubated with 5 μM non-CpG-Cy5 for 90 min and dextran-Alexa Fluor 488 or LysoTracker for last 10 min for the subcellular staining of endosomes and lysosomes, respectively. Confocal microscopy data with differential interference contrast (DIC) images of representative cells are shown. Scale bars, 2.5 μm. Error bars indicate s.d. Data are representative of at least three independent experiments. Figure 1: DNA/RNAs are incorporated into and induce costimulation of CD4 + T cells. ( a ) Naive CD4 + T cells were cultured with indicated TLR ligands (Pam3: 5 μg ml −1 , MALP-2: 5 μg ml −1 , poly(I:C): 100 μg ml −1 , Flagellin: 1 μg ml −1 , Loxoribine: 100 μM, CpG-B: 5 μM) in the presence or absence of immobilized anti-CD3 ∈ Ab (10 μg ml −1 ). After 48-hour incubation, IL-2 production and cell growth were assessed by ELISA and MTS assay, respectively. * P <0.05, Student’s t -test (compared with anti-CD3 alone). ( b ) Naive CD4 + T cells from WT or Myd88 −/− Trif −/− mice were stimulated with the indicated TLR ligands or anti-CD28 (Clone: 37.51, 5 μg ml −1 ) in the presence of immobilized anti-CD3 ∈ Ab. * P <0.05, Student’s t -test (compared with WT cells treated with Pam3). ( c , d ) Naive CD4 + T cells were stimulated with the indicated NAs ( c ) and ODNs ( d ) in the presence of immobilized anti-CD3 ∈ Ab. These T cells were incubated with the Cy5-labelled ODNs at 37 °C for 90 min and ODN uptake was determined by flow cytometry ( d , upper). * P <0.05, Student’s t -test (compared with anti-CD3 alone). ( e ) Naive CD4 + T cells were incubated with 5 μM non-CpG-Cy5 for 90 min and dextran-Alexa Fluor 488 or LysoTracker for last 10 min for the subcellular staining of endosomes and lysosomes, respectively. Confocal microscopy data with differential interference contrast (DIC) images of representative cells are shown. Scale bars, 2.5 μm. Error bars indicate s.d. Data are representative of at least three independent experiments. Full size image We next determined whether this response is mediated by TLRs using mice deficient in both MyD88 and TRIF, which lack the capacity to respond to any of the known TLR ligands. Surprisingly, both poly(I:C) and CpG-B-mediated costimulation were normal in the MyD88/TRIF-doubly deficient CD4 + T cells, whereas MALP-2 (TLR2)-mediated costimulation was completely abrogated ( Fig. 1b ), demonstrating that poly(I:C) and CpG-B-mediated T-cell costimulation was induced independently of TLR signaling. Notably, DNA lacking CpG motifs required for TLR9 activation, such as non-CpG oligodeoxynucleotide (ODN) and DNA encoding GFP (GFP-S and GFP-AS, antisense strand) could also induce costimulation for IL-2 production ( Fig. 1c ). These data indicate that DNA induces T-cell costimulation independently of the CpG motifs. We also found that poly(dA), poly(dC) and poly(dG) but not poly(dT) induced the costimulation for IL-2 production, although the uptake of poly(dT) and non-CpG ODN by T cells was comparable ( Fig. 1d ). Confocal microscopy analysis revealed that non-CpG ODN colocalized with an endosomal marker dextran and a lysosomal marker LysoTracker ( Fig. 1e ), indicating that non-CpG ODN is taken up by T cells and transported to endosomes/lysosomes, similarly in innate cells, and induces costimulatory signals in a TLR-independent manner. Higher-order structure of NA induces T-cell costimulation It is noteworthy that CpG-A possessing a poly(dG)-tail induced stronger costimulation of CD4 + T cells than other ODNs such as CpG-B and non-CpG ( Fig. 1c ). The importance of the poly(dG) tract was confirmed by the finding that control ODN GpC corresponding to CpG-A induces robust IL-2 production, similar to CpG-A ( Fig. 2a ), and that replacement of the poly(dG) motif of GpC by poly(dA), poly(dC) or poly(dT) resulted in the complete loss of stimulatory activity ( Fig. 2b ). 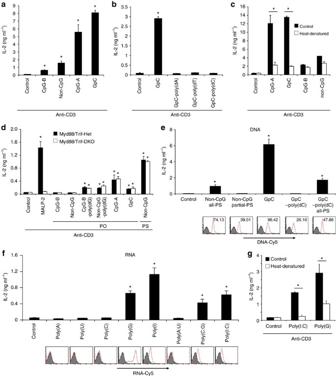Figure 2: Properties of DNA/RNAs required for T cell costimulatory activity. (a–c) Naive CD4+T cells were activated with plate-bound anti-CD3∈with various DNAs—*P<0.05, Student’st-test (compared with anti-CD3 alone) (a); GpC with different poly tails. *P<0.05, Student’st-test (compared with anti-CD3 alone) (b); and heat-denatured ODNs. *P<0.01, Student’st-test (compared with the untreated control) (c). After 48 h, IL-2 production was measured by ELISA. (d) Naive CD4+T cells derived fromMyd88+/−Trif+/−andMyd88−/−Trif−/−mice were activated with immobilized anti-CD3∈together with the indicated DNAs. *P<0.05, Student’st-test (compared with anti-CD3 alone in WT cells). (e) Naive CD4+T cells were stimulated with immobilized anti-CD3∈together with all (all-PS) or partially (partial-PS) PS-modified ODN. CD4+T cells were incubated with the Cy5-labelled ODN at 37 °C for 90 min, washed and analysed for incorporated ODN by flow cytometry (bottom panels). *P<0.05, Student’st-test (compared with anti-CD3 alone). (f) Naive CD4+T cells were stimulated with indicated ODNs and analysed similarly as in (e). *P<0.05, Student’st-test (compared with anti-CD3 alone). (g) Naive CD4+T cells were stimulated and analysed similarly in (c). *P<0.05, Student’st-test (compared with the untreated control). Error bars indicate s.d. Data are representative of at least three independent experiments. Figure 2: Properties of DNA/RNAs required for T cell costimulatory activity. ( a – c ) Naive CD4 + T cells were activated with plate-bound anti-CD3 ∈ with various DNAs—* P <0.05, Student’s t -test (compared with anti-CD3 alone) ( a ); GpC with different poly tails. * P <0.05, Student’s t -test (compared with anti-CD3 alone) ( b ); and heat-denatured ODNs. * P <0.01, Student’s t -test (compared with the untreated control) ( c ). After 48 h, IL-2 production was measured by ELISA. ( d ) Naive CD4 + T cells derived from Myd88 +/− Trif +/− and Myd88 −/− Trif −/− mice were activated with immobilized anti-CD3 ∈ together with the indicated DNAs. * P <0.05, Student’s t -test (compared with anti-CD3 alone in WT cells). ( e ) Naive CD4 + T cells were stimulated with immobilized anti-CD3 ∈ together with all (all-PS) or partially (partial-PS) PS-modified ODN. CD4 + T cells were incubated with the Cy5-labelled ODN at 37 °C for 90 min, washed and analysed for incorporated ODN by flow cytometry (bottom panels). * P <0.05, Student’s t -test (compared with anti-CD3 alone). ( f ) Naive CD4 + T cells were stimulated with indicated ODNs and analysed similarly as in ( e ). * P <0.05, Student’s t -test (compared with anti-CD3 alone). ( g ) Naive CD4 + T cells were stimulated and analysed similarly in ( c ). * P <0.05, Student’s t -test (compared with the untreated control). Error bars indicate s.d. Data are representative of at least three independent experiments. Full size image It has been reported that the poly(dG) tail induces the spontaneous formation of large multimeric aggregates via G-quadruplex formation [15] . Indeed, when GpC was rendered single-stranded by heating and flash-cooling, a dramatic reduction of IL-2 production was observed ( Fig. 2c ), suggesting that higher-order structures mediated by the poly(dG) motif are critical for enhanced costimulation by CpG-A and GpC. Consistently, introduction of a poly(dG)-tail to non-CpG and CpG-B that possess a phosphodiester (PO) backbone sensitive to DNase enabled them to induce costimulation, whereas the same DNA without the poly(dG)-tail could not ( Fig. 2d ). It has been shown that the poly(dG) motif not only protects against DNase degradation [16] but also enhances the cellular uptake of the ODN [17] . Indeed, the uptake of GpC-poly(dC) by T cells was lower than GpC, indicating that GpC-poly(dC) could not induce costimulation due to its poor uptake ( Fig. 2e ). It is noteworthy that cellular uptake of GpC-poly(dC) was weaker than that of non-CpG ( Fig. 2e ). It has been reported that phosphorothioate (PS)-modified ODN are taken up more efficiently than PO-ODN [17] . The entire backbone of non-CpG is PS, whereas it is only partial in GpC ( Supplementary Table 1 ). PS modification of GpC-poly(dC) led to enhanced cellular uptake and costimulation ( Fig. 2e ). By contrast, modification of non-CpG to contain only partial PS resulted in decreased uptake and the failure of costimulation ( Fig. 2e ). We also confirmed that cellular uptake and costimulation of PO-backboned non-CpG was much weaker than those of PS-backboned non-CpG ( Supplementary Fig. 1a ). These data indicate that efficient uptake of DNA via its poly(dG) tail or PS modification is critical for induction of costimulation. While inosine or guanine-containing RNA such as poly(I), poly(G), poly(I:C) and poly(C:G) could induce costimulation, poly(A), poly(U), poly(C) and poly(A:U) could not ( Fig. 2f ). The induction of costimulation by RNA was correlated with the cellular uptake of RNA ( Fig. 2f ). These data indicate that RNA-mediated costimulation depends on the RNA sequence for cellular uptake of RNA to induce costimulation. It has been reported that poly(I) forms parallel four-stranded helices held together by hydrogen-bonded inosine quartets, similar to poly(dG) chains [18] . We found that heat denaturation of poly(I:C) and poly(G) resulted in impaired costimulation ( Fig. 2g ), indicating that the ability of RNA to induce T-cell costimulation is dependent on the higher-order structure similar to DNA. Costimulation induced by NA complexed with LL37 and histones It has been recently shown that endogenous self-DNAs stimulate plasmacytoid dendritic cells by forming aggregated structures upon binding with the antimicrobial peptide LL37 (ref. 19 ). Similarly, we found that mammalian and bacterial genomic DNA were taken up by T cells and induced costimulation when mixed with LL37 while they alone were neither incorporated nor induce stimulation ( Supplementary Fig. 2a , Fig. 3a ). Similarly, although poly(A) and poly(A:U) per se were defective in cellular uptake and induction of costimulation of naive CD4 + T cells ( Fig. 2f ), they were incorporated and induced T-cell costimulation when complexed with LL37 ( Supplementary Fig. 2b , Fig. 3b ). 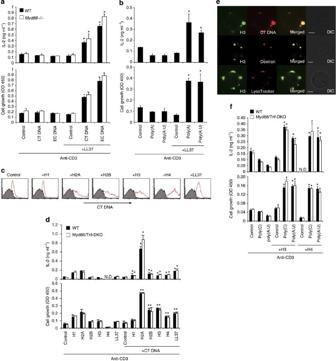Figure 3: T-cell activation by NAs complexed with antimicrobial peptides or core histones. (a,b) Naive CD4+T cells derived from WT andMyd88−/−mice were stimulated with plate-bound anti-CD3∈together with calf thymus (CT)- orE. coli(EC)-derived genomic DNA (a) or RNAs (b) either alone or premixed with LL37. After 48 h, IL-2 production and cell growth were assessed by ELISA and MTS assay, respectively. *P<0.05, Student’st-test (compared with anti-CD3 plus LL37 in WT cells). (c) Naive CD4+T cells were incubated with the Cy5-labelled CT DNA premixed with the indicated histones or LL37 at 37 °C for 90 min and the incorporated DNA were analysed by flow cytometry. (d,f) Naive CD4+T cells derived from WT andMyd88−/−Trif−/−mice were stimulated with plate-bound anti-CD3 together with CT DNA alone (d), RNAs alone (f) or premixed with various histones (d,f), and analysed similarly in (a). *P<0.05, Student’st-test (compared with anti-CD3 plus each histone or LL37 in WT cells). (e) Naive CD4+T cells were stimulated with anti-CD3 with Cy5-labelled CT DNA premixed with Alexa488-labelled histone H3 for 18 h. Endosomes and Lysosomes were visualized by staining with dextran-Alexa Fluor 488 and LysoTracker, respectively. Confocal and differential interference contrast (DIC) images of representative cells are shown. Scale bars, 2.5 μm. Error bars indicate s.d. Data are representative of at least two independent experiments. Figure 3: T-cell activation by NAs complexed with antimicrobial peptides or core histones. ( a , b ) Naive CD4 + T cells derived from WT and Myd88 − / − mice were stimulated with plate-bound anti-CD3 ∈ together with calf thymus (CT)- or E. coli (EC)-derived genomic DNA ( a ) or RNAs ( b ) either alone or premixed with LL37. After 48 h, IL-2 production and cell growth were assessed by ELISA and MTS assay, respectively. * P <0.05, Student’s t -test (compared with anti-CD3 plus LL37 in WT cells). ( c ) Naive CD4 + T cells were incubated with the Cy5-labelled CT DNA premixed with the indicated histones or LL37 at 37 °C for 90 min and the incorporated DNA were analysed by flow cytometry. ( d , f ) Naive CD4 + T cells derived from WT and Myd88 −/− Trif −/− mice were stimulated with plate-bound anti-CD3 together with CT DNA alone ( d ), RNAs alone ( f ) or premixed with various histones ( d , f ), and analysed similarly in ( a ). * P <0.05, Student’s t -test (compared with anti-CD3 plus each histone or LL37 in WT cells). ( e ) Naive CD4 + T cells were stimulated with anti-CD3 with Cy5-labelled CT DNA premixed with Alexa488-labelled histone H3 for 18 h. Endosomes and Lysosomes were visualized by staining with dextran-Alexa Fluor 488 and LysoTracker, respectively. Confocal and differential interference contrast (DIC) images of representative cells are shown. Scale bars, 2.5 μm. Error bars indicate s.d. Data are representative of at least two independent experiments. Full size image Similar to LL37, extracellular histones as components of neutrophil extracellular traps exhibit antimicrobial function [20] . We found that the addition of core histones (H2A, H2B, H3 and H4), but not the linker histone H1, increase cellular uptake of genomic DNA into CD4 + T cells ( Fig. 3c ). The uptake was correlated with induction of costimulation ( Fig. 3d ). Although the genomic DNA–H2A complex was the strongest inducer for IL-2 production, H2A itself induces costimulation in the absence of DNA through unknown mechanism. Therefore, we use H3 that has no costimulatory activity by itself to determine the localization of histone/DNA complexes. The genomic DNA–histone H3 complex was incorporated and localized in endosomes and lysosomes as shown by colocalization with dextran and LysoTracker, respectively ( Fig. 3e ). Similarly to LL37, histone H3 and H4 allowed poly(C) and poly(A:U) to induce costimulation of naive CD4 + T cells ( Fig. 3f ). These data indicated that NAs from self or pathogens could induce T-cell costimulation by forming complexes with antimicrobial peptides such as LL37 or core histones. NA-mediated costimulation is independent of known sensors To determine the mechanism of NA recognition and activation in T cells, we analysed the possible involvement of cytosolic sensors of NAs in innate cells. DNA-dependent activator of IRFs (DAI; also known as ZBP1) was first reported to function as a cytoplasmic DNA receptor [21] . Absent in melanoma 2 (AIM2) was identified as a cytosolic DNA sensor that activates inflammasome [22] . Stimulator of IFN genes (STING) and TBK1 have been identified as essential molecules that mediate a wide range of cytosolic DNA-induced type I IFN responses [23] , [24] , [25] . To examine the possible involvement of these sensors for T-cell costimulation, we tested naive CD4 + T cells derived from Zbp1 −/− , Asc −/− (which links AIM2 to caspase-1), Sting −/− and Tnf −/− Tbk1 −/− mice. However, surprisingly, DNA-mediated costimulation was induced normally in these T cells ( Fig. 4a–c , Supplementary Fig. 3a ), strongly suggesting that T cells utilize a DNA-sensing system different from innate immune cells. 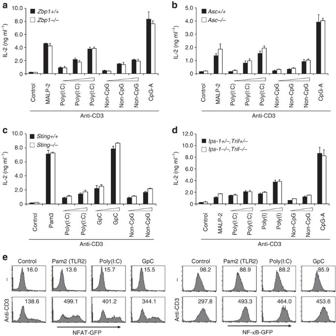Figure 4: NA-mediated T cell costimulation is independent of known innate sensors. (a–d) Naive CD4+T cells derived from WT orZbp1−/−(a),Asc−/−(b),Sting−/−(c) orIps-1−/−Trif−/−(d) mice were stimulated with plate-bound anti-CD3∈and the indicated ligands. After 48 h, IL-2 production was measured by ELISA. (e) T-cell hybridoma reporter cells expressing NFAT-GFP (left) or NF-κB-GFP (right) were stimulated with the indicated ligands with or without immobilized anti-CD3∈for 24 h and analysed by flow cytometry. Error bars indicate s.d. Data are representative of at least two independent experiments. Figure 4: NA-mediated T cell costimulation is independent of known innate sensors. ( a – d ) Naive CD4 + T cells derived from WT or Zbp1 −/− ( a ), Asc −/− ( b ), Sting −/− ( c ) or Ips-1 −/− Trif −/− ( d ) mice were stimulated with plate-bound anti-CD3 ∈ and the indicated ligands. After 48 h, IL-2 production was measured by ELISA. ( e ) T-cell hybridoma reporter cells expressing NFAT-GFP (left) or NF-κB-GFP (right) were stimulated with the indicated ligands with or without immobilized anti-CD3 ∈ for 24 h and analysed by flow cytometry. Error bars indicate s.d. Data are representative of at least two independent experiments. Full size image TLR3 recognizes poly(I:C) in the endosome and initiates signalling through the adaptor, TRIF [1] . On the other hand, retinoic acid-inducible gene I (RIG-I) and melanoma differentiation-associated gene 5 (MDA5) sense poly(I:C) and viral RNA in the cytoplasm, which activates an adaptor, IFN-β promoter stimulator 1 (IPS-1; also known as MAVS) [26] , [27] . To examine the possibility that RIG-I/MDA5 and TLR3 may recognize RNA cooperatively or separately in T cells, we examined RNA-mediated T cell costimulation in IPS-1/TRIF-doubly deficient mice. Normal costimulation by poly(I:C) and poly(I) was observed in Ips-1 −/− Trif −/− T cells ( Fig. 4d ). In addition, to determine the functional redundancy between TLRs and inflammasomes or RIG-I-like receptors (RLRs), we generated MyD88/ASC-and MyD88/IPS-1 doubly-deficient mice. NA-mediated costimulation was normally induced in naive CD4 + T cells from both mutant mice ( Supplementary Fig. 3b,c ). It has been demonstrated that NAs are promiscuously sensed by HMGB proteins to induce type I IFN and pro-inflammatory cytokines [28] . However, downmodulation of all three HMGB proteins in CD4 + T cells using small interfering RNA did not alter IL-2 production in response to NAs ( Supplementary Fig. 3d ). To identify the mechanism underlying the NA-mediated costimulatory signal to induce IL-2 production in T cells, we analysed the activation of NF-κB and NFAT, both of which are essential for T-cell activation [29] . T-cell hybridoma (2B4) expressing the NF-κB-GFP or NFAT-GFP was stimulated by NAs plus anti-CD3. We observed that poly(I:C) and GpC markedly increased activation of NF-κB and NFAT, compared with anti-CD3 alone ( Fig. 4e ). These data suggest that enhanced activation of NF-κB and NFAT is involved in the induction of NA-mediated T-cell costimulation. It is also worth noting that NA-induced costimulation of a T-cell hybridoma, which is definitely free of any innate cells, confirms that NA directly stimulates T cells. NA-mediated costimulation induces Th2 cell differentiation A recent study demonstrated that DNA released from dying host cells stimulates Th2 responses in vivo [30] . It is also reported that stimulation of RLRs by specific ligands biases the immune system toward a Th2 response, whereas the TLR signalling strongly induces Th1 and Th17 responses [31] . Accordingly, it seemed possible that NA-induced stimulation of T cells would induce Th2 cell differentiation. To test this hypothesis, naive CD4 + T cells were stimulated in vitro with anti-CD3 plus anti-CD28 together with various NAs without blocking Abs against IFN-γ or IL-4. NAs such as poly(I:C), poly(I) and non-CpG strongly induced the differentiation of IL-4-producing T cells without the addition of exogenous IL-4 ( Fig. 5a ). By contrast, NAs strongly inhibited the differentiation of IFN-γ-producing T cells ( Fig. 5a ), and also increased the frequency of Th2 cells producing IL-5, IL-9, IL-13 and IL-10 ( Fig. 5a , Supplementary Fig. 4a ). Consistently, the expression of the Th2-master regulator GATA-3 was enhanced, whereas the expression of T-bet, the Th1-master regulator was strongly inhibited in the T cells cultured with NAs ( Supplementary Fig. 4b ), suggesting that NAs directly induce the differentiation of Th2 cells. Notably, unlike NAs, TLR2 ligands had a minimal effect on Th1 and Th2 differentiation ( Fig. 5a ), and NA-mediated costimulation did not affect the development of IL-17-producing T cells ( Supplementary Fig. 4c ). Since NAs induced Th2 differentiation of MyD88/TRIF-double deficient T cells similarly to control T cells ( Supplementary Fig. 4d ), this processes does not require TLR signalling. 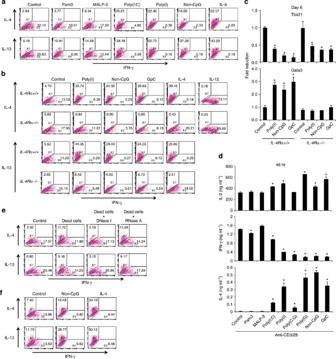Figure 5: NA-mediated costimulation induces Th2 differentiation. (a) Naive CD4+T cells were stimulated with immobilized anti-CD3∈(10 μg ml−1) plus anti-CD28 (10 μg ml−1) and the indicated ligands for 3 days, followed by culture with IL-2 (10 ng ml−1) for an additional 3 days. Cells were subjected to real-time PCR analysis (b), or restimulated with immobilized anti-CD3∈plus anti-CD28 for 6 h for staining of intracellular cytokines IL-4 and IL-13. (b,c) Naive CD4+T cells from WT and IL-4Rα−/−mice were activated similarly as in (a) and cells were subjected to real-time PCR analysis (c) or restimulated with immobilized anti-CD3∈plus anti-CD28 for 6 h for staining of intracellular cytokines IL-4 and IL-13. *P<0.05, Student’st-test (compared with anti-CD3/CD28 plus non-CpG in WT cells). (d) Naive CD4+T cells were stimulated for 48 h with anti-CD3∈plus anti-CD28 and the indicated ligands and cytokine production was analysed by ELISA. *P<0.05, Student’st-test (compared with anti-CD3/CD28 alone). (e) Naive CD4+T cells with or without γ-irradiated naive CD4+T cells (Dead cells) at a 1:1 ratio were stimulated with anti-CD3∈plus anti-CD28 in the presence or absence of DNase I or RNase A, and analysed similarly as in (a). (f) Naive CD4+T cells from OT-II Tg mice were co-cultured with irradiated T cell-depleted splenocytes from C57BL/6 mice as APCs, together with OVA peptide (10 μM) in the presence or absence of non-CpG for 6 days. CD4+T cells were restimulated with immobilized anti-CD3∈plus anti-CD28 for 6 h for staining of intracellular cytokines. Error bars indicate s.d. Data are representative of at least three independent experiments. Figure 5: NA-mediated costimulation induces Th2 differentiation. ( a ) Naive CD4 + T cells were stimulated with immobilized anti-CD3 ∈ (10 μg ml −1 ) plus anti-CD28 (10 μg ml −1 ) and the indicated ligands for 3 days, followed by culture with IL-2 (10 ng ml −1 ) for an additional 3 days. Cells were subjected to real-time PCR analysis ( b ), or restimulated with immobilized anti-CD3 ∈ plus anti-CD28 for 6 h for staining of intracellular cytokines IL-4 and IL-13. ( b , c ) Naive CD4 + T cells from WT and IL-4Rα − / − mice were activated similarly as in ( a ) and cells were subjected to real-time PCR analysis ( c ) or restimulated with immobilized anti-CD3 ∈ plus anti-CD28 for 6 h for staining of intracellular cytokines IL-4 and IL-13. * P <0.05, Student’s t -test (compared with anti-CD3/CD28 plus non-CpG in WT cells). ( d ) Naive CD4 + T cells were stimulated for 48 h with anti-CD3 ∈ plus anti-CD28 and the indicated ligands and cytokine production was analysed by ELISA. * P <0.05, Student’s t -test (compared with anti-CD3/CD28 alone). ( e ) Naive CD4 + T cells with or without γ-irradiated naive CD4 + T cells (Dead cells) at a 1:1 ratio were stimulated with anti-CD3 ∈ plus anti-CD28 in the presence or absence of DNase I or RNase A, and analysed similarly as in ( a ). ( f ) Naive CD4 + T cells from OT-II Tg mice were co-cultured with irradiated T cell-depleted splenocytes from C57BL/6 mice as APCs, together with OVA peptide (10 μM) in the presence or absence of non-CpG for 6 days. CD4 + T cells were restimulated with immobilized anti-CD3 ∈ plus anti-CD28 for 6 h for staining of intracellular cytokines. Error bars indicate s.d. Data are representative of at least three independent experiments. Full size image The generation of Th2 cells is dependent on IL-4–STAT6 signalling, which leads to the upregulation of GATA-3 (ref. 32 ). We assessed whether Th2 differentiation induced by NA-mediated costimulation was also IL-4–STAT6-dependent. IL-4 receptor (R) α-deficient T cells after activation by NAs for 6 days failed to produce any Th2 cytokines including IL-4 and IL-13 ( Fig. 5b ). In addition, the induction of GATA-3 expression was severely diminished in IL-4Rα-deficient T cells ( Fig. 5c ). Similar results were obtained using Stat6 −/− CD4 + T cells ( Supplementary Fig. 4e ), indicating that NA-mediated Th2 differentiation requires IL-4–STAT6 signalling. However, NA-mediated inhibition of IFN-γ production and T-bet expression was still observed in IL-4Rα-deficient T cells ( Fig. 5b,c ), suggesting that NA-mediated inhibition of Th1 differentiation is independent of IL-4 signalling. Therefore, it is likely that NA-mediated costimulation may enhance IL-4 production at an early time point (within 48 h), which then induces Th2 differentiation. Indeed, IL-4 production was induced at 48 h by NAs but not TLR2 ligands, whereas IFN-γ production was reduced ( Fig. 5d ). NA-induced enhancement of IL-2 production was not strong upon stimulation with anti-CD3 plus CD28 as compared with anti-CD3 alone. Strong costimulation with anti-CD28 resulted in reduced enhancement, though significantly enhanced ( Fig. 5d ). Collectively, these data demonstrate that NAs induce Th2 differentiation in an IL-4 signal-dependent manner similarly to the canonical Th2 differentiation pathway induced by exogenous IL-4, whereas suppression of Th1 differentiation by NAs is independent of IL-4 signalling. We next determined whether self-DNA from dead cells induce Th2 differentiation. We found that the addition of dead cells (irradiated naive CD4 + T cells or irradiated HEK 293 cells) to the T-cell culture enhanced the differentiation of IL-4-producing cells, which was cancelled by the addition of DNase I into the medium ( Fig. 5e , Supplementary Fig. 5f ). Addition of RNase A resulted in minimal effect. These data suggest that self-DNA is a critical factor for Th2 differentiation induced by dead cells. To examine whether NA-mediated Th2 differentiation is induced upon antigen stimulation, OVA-specific naive CD4+ T cells from OT-II Tg mice were stimulated with OVA peptide-pulsed irradiated splenocytes plus non-CpG. Non-CpG promoted Th2 differentiation under the condition, strongly suggesting that NAs induces T-cell costimulation even when T cells are activated by antigen-pulsed APCs ( Fig. 5f ). Mechanisms underlying NA-induced Th2 differentiation To determine the mechanism by which NAs induces Th2 differentiation, we compared the gene expression profiles in CD4 + T cells activated under neutral conditions in the presence or absence of non-CpG. Surprisingly, before the upregulation of GATA-3, the expression of T-bet was strongly inhibited by non-CpG-mediated costimulation ( Fig. 6a ). Following the suppression of T-bet expression, the expression of Th2-associated genes was upregulated and IFN-γ was downregulated at 48 h after stimulation ( Fig. 6a ). We further confirmed that various NAs other than non-CpG also induced the suppression of T-bet and the upregulation of GATA-3 and IL-4 expression ( Supplementary Fig. 5a ). We then compared the kinetics of the expression of Th1/Th2-associated genes upon stimulation with IL-4 or non-CpG. GATA-3 was quickly induced in CD4 + T cells by exogenous IL-4 (at 24 h), followed by the induction of Th2 cytokines and the inhibition of T-bet and IFN-γ expression. By contrast, in CD4 + T cells stimulated with non-CpG, GATA-3 expression was induced after inhibition of T-bet expression, suggesting that Th2-associated genes are indirectly induced by non-CpG-mediated costimulation. In addition to these kinetic differences, inhibition of T-bet expression by non-CpG was more rapid and robust than by exogenous IL-4 ( Fig. 6b ). T-bet inhibits Th2 differentiation by directly inhibiting the expression of Th2 cytokines and sequestering GATA-3 from the promoters of Th2 cytokines [33] . Using ChIP analysis, we showed that the binding of GATA-3 to the IL-4 and IL-13 promoters was enhanced in CD4 + T cells by stimulation with non-CpG ( Fig. 6c ). Therefore, it is likely that NA-mediated costimulation induces Th2 differentiation primarily by inhibiting T-bet expression. 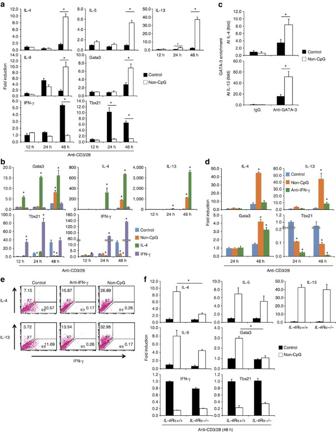Figure 6: Molecular mechanism of NA-mediated Th2 differentiation. (a) Naive CD4+T cells were stimulated with anti-CD3∈plus anti-CD28 with or without non-CpG for the indicated periods and mRNA expression was analysed by real-time PCR. *P<0.01, Student’st-test (compared with anti-CD3/CD28 alone). (b) Naive CD4+T cells were stimulated by NAs or IL-4 and analysed similarly in (a). *P<0.01, Student’st-test (compared with anti-CD3/CD28 alone). (c) Naive CD4+T cells were stimulated with anti-CD3∈plus anti-CD28 together with non-CpG for 48 h, and ChIP analyses were performed by immunoprecipitation with control Ab (IgG) or anti-GATA-3. Quantitative PCR analysis of the GATA3 binding at the IL-4 and IL-13 gene promoters. The results were normalized to those of a standardized aliquot of input chromatin. *P<0.05, Student’st-test (compared with anti-CD3/CD28 alone). (d,e) Naive CD4+T cells were stimulated in the presence of non-CpG or anti-IFN-γ Ab and mRNA expression (d) and intracellular cytokine expression (day 6) (e) were analysed. *P<0.01, Student’st-test (compared with anti-CD3/CD28 alone). (f) Naive CD4+T cells from WT and IL-4Rα−/−mice were stimulated and analysed similarly in (a). *P<0.01, Student’st-test (compared with anti-CD3/CD28 plus non-CpG in WT cells). Error bars indicate s.d. Data are representative of at least two independent experiments. Figure 6: Molecular mechanism of NA-mediated Th2 differentiation. ( a ) Naive CD4 + T cells were stimulated with anti-CD3 ∈ plus anti-CD28 with or without non-CpG for the indicated periods and mRNA expression was analysed by real-time PCR. * P <0.01, Student’s t -test (compared with anti-CD3/CD28 alone). ( b ) Naive CD4 + T cells were stimulated by NAs or IL-4 and analysed similarly in ( a ). * P <0.01, Student’s t -test (compared with anti-CD3/CD28 alone). ( c ) Naive CD4 + T cells were stimulated with anti-CD3 ∈ plus anti-CD28 together with non-CpG for 48 h, and ChIP analyses were performed by immunoprecipitation with control Ab (IgG) or anti-GATA-3. Quantitative PCR analysis of the GATA3 binding at the IL-4 and IL-13 gene promoters. The results were normalized to those of a standardized aliquot of input chromatin. * P <0.05, Student’s t -test (compared with anti-CD3/CD28 alone). ( d , e ) Naive CD4 + T cells were stimulated in the presence of non-CpG or anti-IFN-γ Ab and mRNA expression ( d ) and intracellular cytokine expression (day 6) ( e ) were analysed. * P <0.01, Student’s t -test (compared with anti-CD3/CD28 alone). ( f ) Naive CD4 + T cells from WT and IL-4Rα − /− mice were stimulated and analysed similarly in ( a ). * P <0.01, Student’s t -test (compared with anti-CD3/CD28 plus non-CpG in WT cells). Error bars indicate s.d. Data are representative of at least two independent experiments. Full size image To test this hypothesis further, we compared Th2 differentiation by the blockade of IFN-γ signalling and non-CpG stimulation, because the expression of T-bet is controlled by IFN-γ signalling [34] . We found that the T-bet expression in CD4 + T cells cultured in the presence of anti-IFN-γ was much lower than those stimulated with non-CpG at early time point (48 h) after TCR stimulation ( Fig. 6d ). However, the expression of GATA-3 and Th2 cytokines in T cells cultured with anti-IFN-γ was much lower than those stimulated with non-CpG ( Fig. 6d ), suggesting that inhibition of T-bet expression by non-CpG is not sufficient, though partially contributes, for the upregulation of Th2-associated gene expression. Additional signal(s) are required for the induction of Th2-associated genes by non-CpG-mediated costimulation. Consistently, the Th2 polarization by the presence of anti-IFN-γ was weaker than by non-CpG later (day 6) after TCR priming ( Fig. 6e ). Thus, non-CpG-mediated costimulation simultaneously inhibits T-bet expression and enhances the expression of Th2-associated genes. As T-bet controls Th1 development by directly activating IFN-γ (ref. 34 ), it is likely that NA-mediated costimulation would inhibit Th1 development under Th1-polarizing conditions. As expected, non-CpG inhibits Th1 development and IFN-γ production even under Th1 differentiation condition ( Supplementary Fig. 5b ). We then analysed whether IL-4 signalling is required for the early expression of Th2-associated genes after NA-mediated costimulation. Interestingly, the augmentation of the expression of IL-4 and GATA-3 by non-CpG was severely impaired in IL-4Rα-deficient CD4 + T cells, whereas the upregulation of IL-5, IL-9 and IL-13 expression and downregulation of IFN-γ and T-bet expression was largely unaffected ( Fig. 6f ). Similar results were obtained in the Stat6 −/− CD4 + T cells ( Supplementary Fig. 5c ). These data suggest that non-CpG-mediated T-cell costimulation directly induced the expression of IL-5, IL-9 and IL-13, partly through the inhibition of T-bet expression, whereas IL-4 and GATA-3 expression was induced by IL-4–STAT6 signalling. Naive CD4 + T cells are capable of producing IL-4 upon primary TCR stimulation in the absence of exogenous IL-4, and the early IL-4 is rapidly consumed by the CD4 + T cells themselves [35] . Therefore, NA-mediated IL-4 production may require early IL-4 autocrine signalling to induce the autoactivation of GATA-3 expression. Notably, however, expression of all Th2-associated genes in IL-4Rα-deficient CD4 + T cells disappeared by day 6 after priming with NAs. Although non-CpG stimulation induces the enrichment of GATA-3 on the IL-13 promoter ( Fig. 6c ), it seems that early induction of IL-13 expression by non-CpG (at 48 h) is independent of GATA-3 because IL-13 expression was enhanced by non-CpG in IL-4Rα-deficient CD4 + T cells despite the lack of GATA-3 upregulation by non-CpG ( Fig. 6f ). However, it seems that the enrichment of GATA-3 on the IL-13 promoter is critical for IL-13 expression later (in day 6) after TCR priming for its maintenance because the induction of IL-13 and GATA-3 expression by non-CpG was diminished later after TCR priming (in day 6) in IL-4Rα-deficient CD4 + T cells ( Fig. 5b,c ). These data indicate that autocrine IL-4 is required for the induction of IL-4 and GATA-3 upon non-CpG stimulation, which then acts to amplify and stabilize the expression of Th2-associated genes. The present study shows that NAs directly stimulate CD4 + T cells through a NA sensor different from those of the innate system, subsequently leading to Th2 cell differentiation. In addition to TLRs, a growing number of NA sensors have been identified in the innate immune system, including RLRs, IPS-1-dependent sensors, MyD88/TRIF-dependent sensors, ASC-dependent inflammasomes and STING-dependent sensors [36] . However, we found that recognition of NAs by T cells is independent of all of these known sensors including HMGBs, although we cannot conclusively exclude the possibility that some known NA sensors work redundantly. We found that a higher-order structure of the NAs is required for their incorporation by T cells. Since T cells can incorporate genomic self-DNA only when it is complexed with antimicrobial peptides or core histones, T cells may respond to NAs from dying cells at the site of inflammation and infection, where antimicrobial peptides and/or histones are released. We also demonstrated that specific recognition and uptake of RNA induces costimulatory responses. A recent study demonstrated that cells infected with several viruses including vaccinia virus contained higher-order structured RNA that stimulated MDA5 (ref. 37 ), indicating the possibility that T cells may recognize such viral RNA and are activated. Recent studies demonstrated that, upon infection with nonpermissive HIV, cytoplasmic DNA derived from incomplete reverse transcripts caused CD4 + T cell death through recognition of the cytosolic DNA by a sensor IFI16 followed by activation of the ASC-caspase-1 pathway [38] , [39] . It was also reported that transfected DNA was colocalized with IFI16 in activated T cells [40] . However, our result that DNA-mediated costimulation was normally induced in ASC-deficient CD4 + T cells suggests that IFI16 is not involved in the DNA-mediated costimulation in T cells. While cytosolic DNA stimulates IFI16 upon HIV infection or DNA transfection, incorporated DNAs are accumulated in endosome/lysosome and induce T-cell costimulation in our experiments without activation of IFI16 probably due to the failure to deliver DNA to the cytosol. Furthermore, a recent study showed that immunization with RLR ligands or infection with viruses, which mainly activate RLRs, results in enhanced Th2 responses and much weaker Th1 responses [31] , supporting our observation that NAs directly stimulate the induction of Th2 responses. It is known that TLR stimulation of innate immune cells promotes Th1 and Th17 responses by inducing the Th1-polarizing cytokine IL-12 and the Th17-polarizing cytokines IL-6/IL-23/IL-1 (refs 1 , 41 ). Recent studies, including ours, show that TLR2 ligands directly activate Th1 but not Th2 cells [7] and promote Th17 differentiation [8] . In contrast to TLR, the activation of RLRs suppresses Th1 and Th17 differentiation through the inhibition of IL-12 and IL-23 production, resulting in the enhanced differentiation of Th2 cells [31] . Our results demonstrate that direct stimulation of T cells by NAs strongly inhibit the initial expression of T-bet, which allows the initial production of IL-4 and Th2 cytokines to induce Th2 differentiation. Thus, similar to Th1 and Th17 responses induced by TLRs in innate cells and T cells, it is likely that activation of RLRs in innate cells and the NA sensor in T cells by NAs cooperatively induces Th2 differentiation. The initial origin of IL-4 to trigger Th2 differentiation has been extensively analysed but remains unclear. It has been reported that basophils serve as Th2 cell-promoting APCs by producing IL-4 and/or thymic stromal lymphopoietin [14] . However, their role as APCs remains controversial [42] . It has been suggested that naive T cells are a possible source of IL-4 (refs 43 , 44 ), which modestly induces Th2 differentiation when IFN-γ and IL-12 are neutralized [35] . Although it has been proposed that Th2 differentiation may occur as a default pathway, CD4 + T cells in IL-12 p40-deficient mice fail to differentiate into Th2 cells in response to intracellular pathogens [45] . Thus, the simple blocking of Th1-inducing stimuli such as IL-12 or IFN-γ is not sufficient to induce Th2 differentiation, suggesting the existence of additional Th2-inducing factors. However, such factors for the initial triggering of IL-4 production from naive CD4 + T cells under physiological conditions have not been identified. We here provide strong evidence that the initial IL-4 production derived from naive CD4 + T cells upon recognition of NAs in the absence of any exogenous cytokines or neutralizing antibodies instructs naive CD4 + T cells to differentiate into Th2 cells. A recent report demonstrated that aluminium hydroxide adjuvant (alum) causes cell death and release of host DNA at sites of immunization, which mediates the adjuvant effect for Th2-biased adaptive responses [30] . As the mechanism to induce Th2 responses, it has been reported that uric acid released in the peritoneal cavity after injection of alum may have a role in promoting Th2 cell responses independently of the ASC inflammasome or TLR signalling [46] . As uric acid crystals released at the sites of immunization/inflammation induce extracellular DNA traps formation by neutrophil, eosinophil and basophil [47] , uric acid-induced extracellular DNA traps may directly stimulate T cells to induce Th2 response. A recent study reported that defects in clearance of apoptotic airway epithelial cells upon environmental allergen encounter lead to augmented Th2 cytokine production and airway hyper-responsiveness [48] , indicating that in vivo Th2 responses are closely related to host cell death accompanied by host DNA release. In line with the hypothesis, we found that self-DNA from dead cells induces Th2 differentiation. Collectively, we have identified NAs as a direct Th2-inducing factor, which induces initial production of IL-4 by naive CD4 + T cells, which in turn induces Th2 differentiation. Although we have not identified the NAs sensor in T cells yet, our results provide the possibility that NAs may be critical targets for the development of improved vaccine adjuvants and the overall design of therapeutics to control allergic diseases. Mice C57BL/6 mice were purchased from Clea Japan, Inc. The mice deficient in MyD88, TRIF-deficient, IPS-1 ZBP1 and STAT6 were provided by Dr Akira S. Asc −/− mice were provided by Dr Taniguchi S and Dr Noda T. Sting −/− and Il4ra −/− mice were provided by Dr Barber GN and Dr Brombacher F, respectively. Mice aged 8–16 weeks were used. All mice were maintained under specific pathogen-free conditions and all experiments were conducted under protocols approved by RIKEN Yokohama Institute. ELISA and cell growth analysis Cell culture supernatants were analysed by ELISA for the production of IL-2 (BD biosciences), IL-4 (BD biosciences) and IFN-γ (BD biosciences). Cell growth was assessed by the MTS assay-based Cell Counting Kit-8 (DOJINDO). Helper T-cell differentiation CD4 + /CD25 − /CD62L + /NK1.1 − (naive) T cells were isolated from spleens using a FACS-Aria cell sorter. For Th0 cells, cells were stimulated with plate-bound anti-CD3 (2C11, 10 μg ml −1 ) and anti-CD28 (PV-1, 10 μg ml −1 ) Abs in the presence of the indicated ligands. For Th1 cells, cells were cultured in the presence of IL-12 (10 ng ml −1 ) and anti-IL-4 Abs (10 μg ml −1 ). For Th2 cells, cells were similarly cultured in the presence of IL-4 (10 ng ml −1 ). Real-time quantitative PCR After removal of genomic DNA by treatment with DNase (Wako Nippon Gene), randomly primed cDNA strands were generated with reverse transcriptase II (Invitrogen). RNA expression was quantified by real-time PCR with the following gene-specific primers and values were normalized to the expression of Rps18 mRNA ( Supplementary Table 2 ). Reagents and Abs The TLR2 ligands N -palmitoyl- S -(2,3-bis(palmitoyloxy)-(2 RS )-propyl)-Cys-Ser-Lys 4 (Pam3) and macrophage-activating lipopeptide 2 (MALP-2) were purchased from EMC Microcollections. Poly(I:C), a TLR3 ligand, and LPS ( Escherichia. coli O111:B4), a TLR4 ligand, were obtained from GE Healthcare Biosciences and Sigma, respectively. Flagellin, a TLR5 ligand, and loxoribine, a TLR7 ligand, were obtained from InvivoGen. Oligo DNAs including TLR9 ligands were purchased from Hokkaido System Science. Poly(A), poly(U), poly(C), poly(G), poly(I), poly(A:U) and poly(C:G) were purchased from Sigma. Calf thymus DNA and E. coli DNA was from Sigma and Invivogen, respectively. LL37 was from AnaSpec. Histone H1, H2A, H2B, H3 and H4 were from New England BioLabs. LL37 or histones were first premixed with genomic DNA (peptide:DNA mass ratio of 2:1). After 30-min incubation at room temperature, the mix was added to the T-cell cultures (final concentration was 10 μg ml −1 of DNA). Abs specific for anti-IL-4 PE (11B11, 1:25 dilution) and anti-IFN-γ FITC (XMG1.2, 1:25 dilution) were obtained from BD Biosciences; anti-IL-5 PE (TRFK5, 1:25 dilution), anti-IL-10 PE (1:25 dilution) and anti-IL-13 PE (eBio13A, 1:25 dilution) from eBioscience; anti-IL-9 PE (RM9A4, 1:25 dilution) from BioLegend. ChIP analysis used mAb to GATA-3 (HG3-31AC; Santa Cruz, 1:125 dilution). Intracellular cytokine staining analysis CD4 + T cells were restimulated with immobilized anti-CD3 and anti-CD28 for 6 h in the presence of 2 μM monensin (Sigma, St Louis, MO). Cells were fixed with 4% paraformaldehyde and permeabilized with 0.5% Triton X-100. After blocking with 3% BSA-PBS, cells were stained with antibodies to each cytokine. Flow cytometric analysis was performed on a FACSCalibur and data were analysed with BD CellQuest. Cellular uptake of NA To analyse the uptake of NA, 2 × 10 5 cells were pre-incubated at 37 °C for 10 min in medium. Cells were incubated with fluorescence-labelled NA at 37 °C for 90 min. Then cells were washed once in HANKS/0.1% BSA followed by an acidic wash with 100 mM acetic acid, 150 mM NaCl (pH2.7) for 1 min to remove unbound and cell surface-bound NA. Subsequently, cells were washed two times in HANKS/0.1% BSA, and were analysed by flow cytometry using the FACSCalibur. Reporter cells The 2B4–NFAT-GFP cells have been described [49] and the 2B4-NF-kB-GFP cells were established by transfection of NF-κB-GFP into 2B4 hybridoma cells. These cells were cultured in RPMI 1640 medium supplemented with 10% (vol/vol) FCS and β-mercaptoethanol. Chromatin immunoprecipitation assay Cells were fixed for 10 min at 4 °C with 10% formaldehyde. After incubation, glycine was added to a final concentration of 0.125 M to quench the formaldehyde. Cells were pelleted, washed three times with ice-cold PBS and then lysed. The lysates were sonicated to reduce DNA length to between 200 and 300 base pairs. The chromatin was pre-cleared with protein G agarose beads for 6 h and then incubated with 4 μg of anti-GATA-3 (HG3-31) agarose conjugate antibody (Santa Cruz, sc-268 AC) or control IgG overnight. The precipitates were washed and eluted in 120 μl of NaHCO 3 buffer with 1% SDS. The samples were treated with RNase and Proteinase K and then de-crosslinked at 65 °C overnight. Precipitated DNA was further purified with Qiaquick PCR purification kit (Qiagen) and was analysed by quantitative PCR ( Supplementary Table 2 ) [50] . Confocal microscopic imaging Cells were settled on glass-bottom, 35-mm tissue culture dishes (MATSUNAMI GLASS). Confocal microscopy analyses were performed with a Leica TCS SP5 confocal microscope with an oil immersion objective (HCX PL APO × 63/1.40–0.60 NA, Leica). Dual-color images were acquired using a sequential acquisition mode to avoid cross-excitation. To visualize the Histone–calf thymus DNA complex in CD4 + T cells, calf thymus DNA (Sigma) was labelled with Cy5 using the Label IT Nucleic Acid Labelling Reagents (Mirus) and histone H3 was labelled with DyLight 488 using the antibody labelling kit (Pierce), according to the standard protocol provided by the respective manufacturers. RNA interference Double-stranded oligonucleotides corresponding to the target sequences were cloned into the pSuper.Retro RNAi plasmid (OligoengineInc.). The siRNA targeting sequences which function for commonly all three murine HMGB1/2/3 are 5′-GAGAAGTATGAGAAGGATATT-3′ and 5′-AAGTATGAGAAGGATATTGCT-3′. Statistics Statistical significance was determined by a two-tailed unpaired Student’s t -test. P <0.05 was considered statistically significant. How to cite this article: Imanishi, T. et al. Nucleic acid sensing by T cells initiates Th2 cell differentiation. Nat. Commun. 5:3566 doi: 10.1038/ncomms4566 (2014).